Contribution of Arctic seabird-colony ammonia to atmospheric particles and cloud-albedo radiative effect The Arctic region is vulnerable to climate change and able to affect global climate. The summertime Arctic atmosphere is pristine and strongly influenced by natural regional emissions, which have poorly understood climate impacts related to atmospheric particles and clouds. Here we show that ammonia from seabird-colony guano is a key factor contributing to bursts of newly formed particles, which are observed every summer in the near-surface atmosphere at Alert, Nunavut, Canada. Our chemical-transport model simulations indicate that the pan-Arctic seabird-influenced particles can grow by sulfuric acid and organic vapour condensation to diameters sufficiently large to promote pan-Arctic cloud-droplet formation in the clean Arctic summertime. We calculate that the resultant cooling tendencies could be large (about −0.5 W m −2 pan-Arctic-mean cooling), exceeding −1 W m −2 near the largest seabird colonies due to the effects of seabird-influenced particles on cloud albedo. These coupled ecological–chemical processes may be susceptible to Arctic warming and industrialization. Over the past 50 years, the Arctic has been warming more rapidly than the global-mean rate for the Earth [1] . Atmospheric particles, clouds and their interactions play key, but complex, roles in offsetting a substantial portion of the Earth’s global-mean radiative forcing from greenhouse gases [2] , yet contribute the largest uncertainty to the total radiative forcing estimate [1] . Within the Arctic climate system there are many delicately balanced inter-connections between processes related to the land, ice, ocean and atmosphere [2] , [3] , [4] , [5] , [6] , [7] . The Arctic is a challenging region to model [6] , although skill and process understanding is progressing [3] , [5] , [7] . In this study, we present and investigate a previously unknown coupling between migratory Arctic seabirds and cloud radiative effects ( Fig. 1 ). This climate coupling occurs through changes in atmospheric particle number in response to seabird-colony ammonia (NH 3 ). 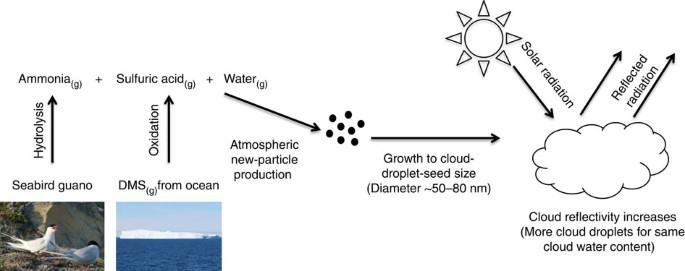Figure 1: Seabird–climate coupling. Schematic summary of processes that couple Arctic seabird-colony ammonia emissions with climate. Figure 1: Seabird–climate coupling. Schematic summary of processes that couple Arctic seabird-colony ammonia emissions with climate. Full size image Together with gas-phase sulfuric acid (H 2 SO 4 ) and water, NH 3 can form new particles in the atmosphere with diameters of ∼ 1–2 nm (refs 8 , 9 , 10 ) that can continue to grow to sizes that affect climate [11] , [12] , [13] . This particle formation process is widely accepted as a key contributor to particle number in the Earth’s troposphere, with particle formation rates being highly sensitive to NH 3 mixing ratios between about 1 and 100 p.p.t.v. (parts per trillion by volume; ref. 8 ). If newly formed particles grow by condensation of sulfuric acid, organic vapours and/or other compounds to diameters larger than ∼ 50–80 nm, they could influence climate indirectly by acting as the seeds for cloud-droplet formation, modifying the reflectance of solar radiation by clouds [11] , [12] , [13] . More abundant particles form more-numerous and smaller cloud droplets for a fixed cloud liquid-water content, that in turn increase cloud reflection of solar radiation; a cooling effect [12] . The impact of NH 3 emissions from Arctic summertime seabird guano on particle formation and cloud radiative effects has not been previously identified or quantified, and despite the known importance of NH 3 for particle formation, there are few NH 3 measurements in the Arctic [14] , [15] , [16] . In the summertime Arctic, the precursor vapours for particle formation arise from natural local sources [3] , [17] , [18] , [19] . Natural H 2 SO 4 arises from oxidation of dimethyl sulfide (DMS) that is produced by marine biological activity. Wind facilitates the transfer of DMS from the ocean into the atmosphere, where oxidation produces sulfur dioxide (SO 2 ). Ultimately, H 2 SO 4 is produced either through SO 2 aqueous oxidation in clouds or in the gas phase by reaction of SO 2 with atmospheric oxidants. Only the latter of these oxidation pathways leads directly to particle formation that increases particle number. Bacterial hydrolysis of seabird guano produces NH 3 (ref. 20 ), previously linked to particle formation in remote regions downwind of penguin colonies [21] . In the Arctic and near-Arctic regions north of 50° N, recent emission inventories suggest that migratory seabird colonies emit about 40 Gg of NH 3 each year [18] , [19] , primarily between May and September when some tens of millions of breeding pairs are nesting in the region. Several recent global chemical-transport model (CTM) studies have implemented these or similar seabird-colony NH 3 emissions [7] , [14] , [22] , although none have investigated the impact of these emissions on size-resolved particle number concentrations, clouds and climate as depicted in Fig. 1 . The oceans contribute a relatively smaller amount to Arctic summertime NH 3 emissions [22] and have been identified as a net sink of NH 3 in the summertime Canadian Arctic Archipelago [14] . Other particle-precursor vapours of natural origin, which we consider later in our discussion, include extremely low-volatility organic compounds (EL-VOCs), amines and iodine [23] , [24] , [25] , [26] . Wentworth et al . [14] recently measured summertime atmospheric surface-layer NH 3 mixing ratios during a 2014 shipboard campaign in the Arctic as part of a multi-year research project (NETCARE, NETwork on Climate and Aerosols: addressing key uncertainties in Remote Canadian Environments; ‘Methods’ section) and presented evidence that seabird colonies are significant sources of NH 3 in the summertime Arctic. Wentworth et al . [14] also showed that observed summertime PM 1.0 (particulate matter with diameters smaller than 1.0 μm) in the high Arctic at Alert, Nunavut, Canada are significantly more neutralized (indicating the availability of gas-phase NH 3 ) than during the rest of the year, when previous aircraft measurements have also indicated Arctic aerosol to be highly acidic [27] . However, the influence of seabird-colony NH 3 on particle formation, particle number concentrations and cloud-albedo radiative forcing ( Fig. 1 ) has not yet been examined. In this study, we quantify particle-number changes and the particle-induced cloud-albedo radiative effect in response to Arctic seabird-colony ammonia emissions. We use the GEOS-Chem-TOMAS (GCT) CTM [7] , [28] , [29] with online aerosol physics and chemistry (‘Methods’ section and Supplementary Methods ) to quantify the impact of seabird-colony NH 3 emissions on Arctic atmospheric surface-layer reduced nitrogen (gas-phase NH 3 and particulate ammonium (NH 4 + )), particle formation, growth and subsequent radiative impacts of particle-induced modification of cloud properties. GCT is a state-of-the-science model for this application as it includes the chemical and physical pathways that connect NH 3 emissions to climate through particle formation and condensational growth, balanced by losses due to gas and particle scavenging, both in and below clouds. Our results show that ammonia from Arctic seabird-colony guano makes a key contribution to bursts of newly formed particles that are observed in the summertime Arctic. Our simulations indicate that growth of these seabird-influenced particles yield pan-Arctic-mean cooling tendencies that could be large (about −0.5 W m −2 ) due to particle-induced changes in cloud albedo. This climate-relevant coupling between Arctic seabirds and cloud radiative effects is explored in the following sections. 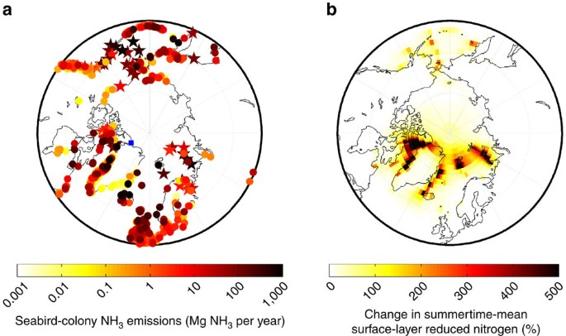Figure 2: Arctic seabird-colony NH3(g)emissions and impacts on atmospheric surface-layer NH3(g)and NH4+(p)mixing ratios. (a) Locations and annual emissions of NH3(g)from Arctic seabird colonies. Circles indicate colonies in the Riddicket al.18,19inventory and stars are additional colonies from the Circumpolar Seabird Data Portal30. The blue square shows the location of Alert, Nunavut, Canada. (b) Percent change in summertime mean atmospheric surface-layer total reduced nitrogen (gas-phase ammonia (NH3(g)) and particulate ammonium (NH4+(p))) attributed to the seabird-colony NH3emissions for the GEOS-Chem-TOMAS simulations. Atmospheric reduced nitrogen from Arctic seabird guano Figure 2a shows the geographic distribution of total annual Arctic seabird-colony NH 3 emissions from recent inventories [18] , [19] , [30] that were implemented in our GEOS-Chem-TOMAS simulations between the months of May and September. Further details about these NH 3 emissions are provided in the ‘Methods’ section. Figure 2b shows that in the majority of the ice-free Arctic, the seabird-colony emissions yield a 50–500% increase in the simulated summertime atmospheric surface-layer total reduced nitrogen (gas-phase NH 3 and particulate NH 4 + ) relative to a simulation without the seabird-colony NH 3 emissions. For these simulations, 61% of the Arctic atmospheric surface layer pole-ward of 66° N increases in NH 3 by more than 50%. This highlights the pan-Arctic potential for seabird-guano NH 3 to increase particle formation. The seabird-colony-reduced nitrogen source accounts for about 40% of the simulated summertime surface-layer total reduced nitrogen and 90% of the NH 3 in the Canadian Arctic Archipelago region north of 70° N. Wentworth et al . [14] found that GEOS-Chem-simulated NH 3 near Alert was at the lower limit of the range of shipboard measurements, suggesting the Arctic seabird source may be even larger or there may be other unidentified sources. Model-measurement comparisons along the NETCARE ship track in the Canadian Arctic Archipelago region indicates that Arctic seabird-colony emissions can produce NH 3 mixing ratios of 10 to 1,000 p.p.t.v., whereas without those emissions, NH 3 mixing ratios are underestimated by two to three orders of magnitude in the GEOS-Chem CTM [14] ( Supplementary Figs 1 and 2 ). Figure 2: Arctic seabird-colony NH 3(g) emissions and impacts on atmospheric surface-layer NH 3(g) and NH 4 + (p) mixing ratios. ( a ) Locations and annual emissions of NH 3(g) from Arctic seabird colonies. Circles indicate colonies in the Riddick et al . [18] , [19] inventory and stars are additional colonies from the Circumpolar Seabird Data Portal [30] . The blue square shows the location of Alert, Nunavut, Canada. ( b ) Percent change in summertime mean atmospheric surface-layer total reduced nitrogen (gas-phase ammonia (NH 3(g) ) and particulate ammonium (NH 4 + (p) )) attributed to the seabird-colony NH 3 emissions for the GEOS-Chem-TOMAS simulations. Full size image Arctic aerosol neutralization as evidence of ammonia levels We consider the weekly aerosol neutralization measurements [14] conducted using filter samples at Alert, Nunavut, Canada as evidence of NH 3 levels since there are no ongoing NH 3 measurements at Alert. We conduct thermodynamic calculations to estimate the summertime NH 3 mixing ratios indicated by the ion concentrations in the Alert aerosol filter measurements (‘Methods’ section and Supplementary Fig. 3 ). Our thermodynamic calculations indicate that NH 3 mixing ratios above 1 p.p.t.v. (and plausibly as high as 1 p.p.b.v.) are consistent with the summertime measurements at Alert that show the aerosol neutralization ratio typically exceeds 0.7 ( Supplementary Fig. 4 ). These levels of NH 3 are consistent with the NH 3 mixing ratios measured during the 2014 NETCARE-shipboard campaign [14] . GEOS-Chem simulations indicate that Arctic seabird-colony NH 3 emissions provide sufficient NH 3 to contribute the majority of these NH 3 levels [14] . Outside of summer, the aerosol neutralization ratio based on Alert filter measurements is typically less than 0.4, and our calculations indicate that this corresponds to NH 3 levels of less than 1 p.p.t.v. This annual cycle in the particle neutralization state occurs each year and also suggests that seabird-colony emissions are a key source of the NH 3 since the timing of the greatest neutralization in the observations coincides with the period of the migratory seabird-colony emissions. 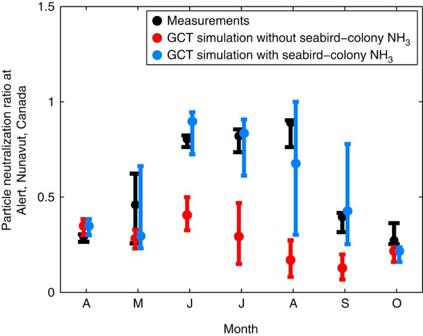Figure 3: Aerosol neutralization state at Alert. Monthly median (April to October) aerosol neutralization ratios from filter measurements (black) at Alert, Nunavut, Canada and for the GEOS-Chem-TOMAS (GCT) simulations with (blue) and without (red) seabird-colony NH3emissions. Error bars show the 20th and 80th percentiles. Figure 3 shows that implementation of the seabird-colony NH 3 source into the GCT model is sufficient to yield the summertime maximum in aerosol neutralization state at Alert in the GCT simulations. This change increases the simulated monthly median aerosol neutralization ratio from about 0.4 to about 0.9 over June–August in our GCT simulations. Implementation of the seabird-colony emissions into GCT reduces the model-measurement summertime mean fractional bias [31] in neutralization state from +1.0 to +0.1. Consideration of methane sulfonic acid (MSA) changes the neutralization ratio at Alert by about 0.05 or less in all months, with the greatest effect in August. Figure 3: Aerosol neutralization state at Alert. Monthly median (April to October) aerosol neutralization ratios from filter measurements (black) at Alert, Nunavut, Canada and for the GEOS-Chem-TOMAS (GCT) simulations with (blue) and without (red) seabird-colony NH 3 emissions. Error bars show the 20th and 80th percentiles. Full size image Role of Arctic seabird-colony ammonia in particle formation Each summer, bursts of particles with diameters larger than 10 nm (N10) are observed at Alert [4] . 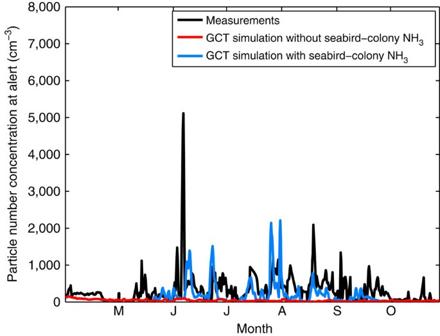Figure 4: Summertime bursts of newly formed particles at Alert. Time series of surface-layer number concentration of atmospheric particles larger than 10 nm (N10) from condensation particle counter (CPC) measurements at Alert from April to October 2011 (black) and as simulated with GCT model, with (blue) and without (red) seabird emissions implemented. Figure 4 shows the time series of the measured N10 particle number concentration from the condensation particle counter at Alert (‘Methods’ section). Scanning mobility particle sizer (SMPS) measurements (Methods) indicate that these summertime N10 spikes are dominated by particles with diameters smaller than 20 nm, rather than larger accumulation-mode particles that are often associated with long-range transport. In the summertime, the Arctic atmosphere reaches its most pristine state owing to efficient cleaning by precipitation [5] , [6] , [7] , [32] , [33] , [34] , which favours particle formation since available vapours are more likely to form new particles because the surface area for condensation on existing particles is reduced by precipitation in low clouds. Figure 4: Summertime bursts of newly formed particles at Alert. Time series of surface-layer number concentration of atmospheric particles larger than 10 nm (N10) from condensation particle counter (CPC) measurements at Alert from April to October 2011 (black) and as simulated with GCT model, with (blue) and without (red) seabird emissions implemented. Full size image Next, we use the GCT model to assess the role of the extra NH 3 from Arctic seabird guano in the observed summertime N10 bursts at Alert. Using a state-of-the-science ternary (NH 3 +H 2 SO 4 +H 2 O) particle formation scheme [35] , [36] (‘Methods’ section), the GCT model more-closely simulates these N10 bursts when the seabird-colony NH 3 source is implemented relative to an otherwise similar simulation without this NH 3 source ( Fig. 4 ), reducing the mean-fractional bias [31] relative to measurements from −0.86 to −0.47. The timing and magnitude of the N10 bursts is reasonably well represented with the GCT model, but inconsistencies may arise because the seabird-colony emissions are emitted uniformly between May and September and potential sub-grid scale effects related to plume dispersion of seabird-colony NH 3 are not considered. Previous studies have found a variety of trace gases including amines [9] , [37] , EL-VOCs [23] , [24] , [25] and iodine [26] that could also stabilize nascent particles. We considered whether they could contribute to additional particle formation near Alert. During the NETCARE 2014 summertime shipboard campaign near Alert, gas-phase amines were consistently below the instrument detection limit of 0.5 p.p.t.v. (‘Methods’ section and Supplementary Table 1 ). These low concentrations of amines might enhance particle formation [9] , but in contrast, gas-phase ammonia observations during NETCARE 2014 ranged from 40 to 870 p.p.t.v., which are levels typically associated with significant particle formation and early growth. If amines did participate in particle formation, this would need to be very close to their source, before the gas-phase amines condense on pre-existing particles or react with gas-phase oxidants. Previous studies indicate lower concentrations of EL-VOCs in the Arctic than needed to fully support the observed particle formation [24] , [38] . We conducted calculations of the expected contribution from EL-VOC-related particle formation in this region based on current knowledge of EL-VOC sources (‘Methods’ section) and found a low contribution. Iodine oxides have also been linked to particle formation in Arctic coastal regions [26] . The spatial extent of this influence is not well established. We have no observational constraints on the gas-phase iodine oxides near Alert, so we cannot rule out their additional contributions (‘Methods’ section). Primary marine aerosols can also contribute to the number of ultrafine particles in certain regions of the Arctic [39] , [40] , [41] , [42] , which could regionally reduce the relative contribution of seabird-colony emissions to ultrafine particle number concentrations. On the other hand, MSA can contribute to particle formation if a base exists for the nascent clusters [43] , [44] , and as a result could increase the relative contribution of seabird-colony emissions to the number of ultrafine particles. However, recent evidence by Giamarelou et al . [15] suggests that ammonium sulfate is the dominant constituent in sub-12 nm particles near the high-Arctic site Ny-Ålesund, Svalbard. This supports our use of the particle-formation scheme based on ammonia, sulfuric acid and water. Given that current knowledge about particle-formation processes is limited, possibly NH 3 may act along with other co-emitted trace gases and in concert with MSA in yielding the observed N10-particle bursts at Alert. We consider all of the above together as compelling evidence for the key role of seabird-colony emissions in Arctic particle formation and early growth. Seabird-influenced particle growth to cloud-relevant size To influence clouds and radiation, the nascent particles must grow to sizes larger than ∼ 50–80 nm; sizes that act as the seeds for cloud-droplet formation in summertime Arctic clouds [4] , [12] , [13] . Our GCT simulations indicate sufficient growth of the seabird-colony-influenced particles that the number of particles larger than 80 nm (N80) increases throughout the summertime Arctic surface layer by 10–50% over most of the Arctic Ocean, with the largest changes near the major seabird colonies, particularly in the Canadian Arctic Archipelago region, and also along the eastern coast of Greenland, towards Iceland ( Supplementary Fig. 5 ). The simulated pan-Arctic-mean surface-layer N80 for August increased from 40.4 to 49.5 cm −3 with the implementation of seabird-colony NH 3 . Thus, there is sufficient growth of the newly formed particles associated with the extra NH 3 from seabird colonies to yield pan-Arctic changes in the number of particles that are large enough to potentially act as the seeds for the formation of cloud droplets. As well, with the seabird-colony ammonia implemented, the simulated regional-mean surface-layer number of cloud-condensation nuclei (CCN) at 0.2% supersaturation (CCN0.2) over the pack ice of the inner Arctic Basin for August is about 18 cm −3 , which is within the range of measurements from the region [3] (15–30 cm −3 ; ‘Methods’ section and Supplementary Fig. 6 ). Without this ammonia source and for the same region, the simulated regional-mean surface-layer CCN0.2 for August is 12 cm −3 and the CCN0.2 is less than 10 cm −3 over much of the pack ice region of the inner Arctic, which underestimates the measurements [3] . Over the inner Arctic (north of 80 °N), the simulated summertime regional-mean CCN0.2 concentrations are most sensitive to the extra ammonia source at altitudes below about 1.2 km (changes of about 20–30%; Supplementary Fig. 7 ). This suggests that the greatest impacts of the seabird-colony ammonia are on clouds in the lower troposphere. The simulated CCN0.2 concentrations decrease from 500 m to the surface layer ( Supplementary Fig. 7 ), as do measurement vertical profiles from this region [45] . This decrease towards the surface is thought to be due to efficient particle removal in and below low-level clouds combined with limited mixing into the stable surface layer of air that originates near particle sources (open water, land), rises and is transported into the inner Arctic above the surface layers [3] . Condensation of sulfuric-acid and low-volatility organic vapours contributes to particle growth in our simulations. Sulfate and organic carbon account for about 70 and 30%, respectively, of the simulated mass of particles with diameters of about 80 nm. There is considerable uncertainty about primary organic aerosol and low-volatility organic-vapour precursor emissions from the oceans [17] . Thus, our simulations, while exhibiting skill in representing Arctic particle number and size distributions [7] , may miss additional particles and vapours that could enhance particle number and growth. 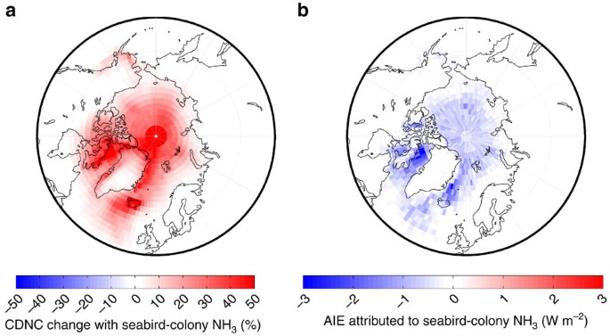Figure 5: Pan-Arctic geographic distribution of climate components of the seabird–climate coupling. (a) Percent difference in pan-Arctic summertime mean cloud-droplet number concentration (CDNC) in the atmospheric boundary layer due to inclusion of seabird NH3emissions in the GEOS-Chem-TOMAS (GCT) model under the assumption of fixed cloud liquid-water content. (b) Pan-Arctic summertime-mean aerosol indirect (cloud-albedo) radiative effect (AIE) attributed to the seabird-colony emissions. Seabird-influenced cloud-droplet number concentration change Figure 5a shows that implementation of seabird-colony emissions in the GCT model increases simulated pan-Arctic cloud-droplet number concentrations (CDNCs) by over 10% through most (64%) of the Arctic boundary layer under the assumption of fixed cloud liquid-water content. Maximum changes exceed 50% in close proximity to the larger seabird colonies. The simulated aerosol activation treatment is described in the ‘Methods’ section, including details about the supersaturation and particle size that activates ( Supplementary Figs 8 and 9 ). The simulated CDNC is broadly consistent with the measurements of Leaitch et al . [46] made during the summertime 2014 NETCARE campaign in the Canadian Arctic Archipelago region ( Supplementary Fig. 10 ). Leaitch et al . [46] found a median CDNC of 10 and 100 cm −3 for clouds below and above 200 m, respectively. Our simulated CDNC falls within that general range, albeit with a weaker, but similar, vertical gradient. The agreement with these recent measurements [46] gives confidence in the simulation of CDNC. Next we investigate the cloud-albedo radiative effect under the assumption of fixed cloud liquid-water content. Figure 5: Pan-Arctic geographic distribution of climate components of the seabird–climate coupling. ( a ) Percent difference in pan-Arctic summertime mean cloud-droplet number concentration (CDNC) in the atmospheric boundary layer due to inclusion of seabird NH 3 emissions in the GEOS-Chem-TOMAS (GCT) model under the assumption of fixed cloud liquid-water content. ( b ) Pan-Arctic summertime-mean aerosol indirect (cloud-albedo) radiative effect (AIE) attributed to the seabird-colony emissions. Full size image More-numerous and smaller cloud droplets (for the same cloud liquid-water content) make clouds more reflective of solar radiation, which has a cooling effect [11] , [12] , [13] . Here we restrict our investigation to this single aerosol–cloud radiative effect. Further study is needed to consider additional particle-induced cloud-albedo radiative effects related to changes in cloud lifetime, liquid-water content and fractional coverage, which might be particularly relevant in summertime in the pristine region north of about 80–85° N (ref. 47 ). In addition, longwave radiative effects associated with cloud-property changes in response to particle number might be relevant in the low-CDNC limit, particularly in the near-surface layers over the inner Arctic north of about 80–85° N where the clouds are not optically thick with respect to longwave radiation [47] . Observations show that Arctic low-cloud layers further above the surface layer ( ∼ 200–500 m and above) tend to have greater cloud droplet number concentrations [46] for which longwave radiative effects are relatively insensitive to changes in particle number [47] . However, future study is needed to examine the longwave effects of seabird-colony ammonia, particularly in the inner Arctic and as well to develop understanding of processes controlling aerosol activation to form cloud droplets in this region. Cloud-albedo radiative effect attributed to seabird ammonia We conduct an offline calculation of the cloud-albedo radiative effect in response to changes in particle number under constant cloud water content [12] , [48] , [49] (‘Methods’ section). The mean aerosol indirect effect (AIE) over the Arctic Ocean between our simulations with and without the extra seabird-colony NH 3 is −0.5 W m −2 , and exceeds −1 W m −2 near the largest bird colonies ( Fig. 5b ). We find no appreciable change in the direct scattering and absorption related to these additional particles because the particle mass concentrations do not change greatly between simulations, and the size distribution shifts only slightly at the sizes with most-efficient scattering ( Supplementary Methods ). In the context of current global radiative forcing from CO 2 (+1.6 W m −2 ; ref. 50 ), the negative contribution from the Arctic seabird-influenced cloud-albedo radiative effect is a significant regional effect. Future work is needed to fill knowledge gaps related to seabird-colony NH 3 emissions, the role of MSA, primary organic particles from the oceans and secondary organic aerosols from both marine and terrestrial sources in shaping Arctic particulate mass and number distributions and also cloud processes (cloud formation, growth and lifetime), particularly in the inner Arctic. We conducted sensitivity studies, which show the cloud-albedo radiative effect could be both strengthened and weakened by these processes (‘Methods’ section and Supplementary Table 2 ). Our findings suggest that the pristine summertime Arctic is an environment where changes in particle formation can have a noteworthy impact on cloud radiative effects. Here, we have investigated the contribution of seabird-colony ammonia emissions to Arctic particle-number concentrations and identified a resultant substantial cloud-albedo radiative effect in response to changes in cloud-droplet number for fixed cloud liquid-water content. The evidence that migratory seabirds are a major source of NH 3 in the Arctic and a key contributor to Arctic particle formation draws attention to the connections between the fauna, nitrogen cycle, atmospheric aerosol and aerosol–cloud interactions in the Arctic. Our study highlights the need for multi-disciplinary research, ongoing measurements of NH 3 , particles and clouds in the Arctic region, and detailed study of the natural Arctic fauna to better understand the details of the related processes. Given the accelerated rate of Arctic warming [1] , [2] , [51] , seabird numbers and migratory patterns may change, altering the seabird-guano NH 3 emissions in the Arctic. Climate warming may also change other particle sources in the Arctic through oceanic emissions [52] , [53] , ship traffic [54] and other anthropogenic pollution. Thus, the relative importance of NH 3 from seabird guano to the Arctic climate may be susceptible to future change. Shipboard trace-gas measurements Measurements of gas-phase NH 3 were taken in the Canadian Arctic Archipelago region aboard the Canadian Coast Guard Ship (CCGS) Amundsen during a NETCARE (NETwork on Climate and Aerosols: addressing key uncertainties in the Remote Canadian Environments) campaign from 13 July 2014 to 7 August 2014 (ref. 14 ). The measurements were conducted in Baffin Bay, Lancaster Sound and Nares Strait. NH 3 was quantified using the Ambient Ion Monitor-Ion Chromatograph (AIM-IC) system (Model 9000D, URG Corp.). The AIM-IC is a semi-continuous, on-line instrument that provides hourly measurements of both water-soluble gases and ions in particulate matter with a diameter smaller than 2.5 μm (PM 2.5 ). Ambient air is pulled through a parallel plate wet denuder, which scavenges water-soluble gases, whereas PM 2.5 are collected downstream in a supersaturation chamber. These aqueous samples are then quantified in an online manner using both an anion and cation Ion Chromatograph (ICS-2000, Dionex Corp.). IC calibration was performed offline with aqueous standards, and a system background was determined by overflowing the inlet with zero air (AI 0.0 UZ-T, PraxAir). An NH 3 detection limit of 38 p.p.t.v. was calculated by taking 3σ of the background signal. To prevent influence from activities aboard the ship, NH 3 measurements are only reported if the following conditions were met: ship speed >4 knots, apparent hourly wind direction ±90° of the bow (where the inlet box containing the denuder and supersaturation chamber was located), and standard deviation of apparent wind direction <36°. Detection limits for six different amines during this study are given in Supplementary Table 1 and were determined in a similar manner to NH 3 . The instrumental backgrounds for amines are very low and there was no signal from any amine listed in Supplementary Table 1 during the zero air experiments conducted throughout the NETCARE 2014 shipboard campaign. As a result, we calculate the detection limits by taking three times the minimum peak area that can be integrated and convert this to either a mixing ratio (gas-phase) or mass loading (PM 2.5 ). Not once throughout the entire study did any amine exceed the detection limit. Thus, we did not find clear indications in the study region near Alert that the amines typically associated with particle formation (particularly dimethylamine) were available at levels typically associated with significant particle formation [9] , although particle formation could have occurred very near to source before loss to particle phase or further gas-phase oxidation reactions. Iodide (I − ) in PM 2.5 and gas-phase hydrogen iodide (HI) can also be detected by the AIM-IC. Detection limits of 18 ng m −3 and 0.7 p.p.t.v. were calculated for I − and HI, respectively. Similar to the amines, neither I − nor HI was observed above the detection limit during the NETCARE 2014 shipboard campaign. Unfortunately, we have no measurements of iodine oxides in the Alert region, such that we cannot rule out their potential additional contributions to particle formation, particularly as iodine has been linked to particle formation in certain coastal regions [26] . Thus, while the potential exists for amines and iodine to make additional contributions to particle formation in our study region, we were unable to ascertain their influence from available measurements, whereas we have clear evidence of NH 3 at levels known to strongly influence particle formation and early growth. We recommend future study of the composition of nascent aerosol clusters in the Arctic to address these uncertainties. Alert particle measurements and thermodynamic calculations Particle size distribution measurements at Alert have been ongoing since March 2011 (ref. 4 ). The total number concentration of particles with diameters larger than 10 nm at Alert is measured with a TSI 3772 Condensation Particle Counter (CPC). The 3772 CPC was initially compared with a TSI 3775 CPC, which counted particles larger than 4 nm and was operating temporarily at the site, and the differences were found to be <10% when particle sizes were large enough such that both counters counted all the particles. The particle size distributions from 20 to 500 nm diameter are measured with a TSI 3034 Scanning Mobility Particle System (SMPS), verified for sizing on site using mono-disperse particles of polystyrene latex and of ammonium sulfate generated with a Brechtel Manufacturing Incorporated Scanning Electrical Mobility Spectrometer, and for number concentrations through comparison with the TSI 3772 Condensation Particle Counter (CPC). The 3772 CPC also compares to within 10% with SMPS when particle sizes are large enough for all the particles to be counted by both the instruments. In addition, weekly samples of the ambient aerosol are collected on Teflon filters located inside the Global Atmosphere Watch (GAW) Observatory at Alert. The sampling uses a cyclone to restrict te particles to smaller than 1 μm. Ion chromatography is conducted for the analysis of major inorganic ions (including SO 4 2− , NH 4 + and NO 3 − ) and MSA. Further details about the sample handling, analytical methods and quality control are discussed by Leaitch et al . [4] and Li and Barrie [55] . There are no ongoing measurements of NH 3 at Alert. In addition, since the particle composition measurements at Alert are based on integrated weekly filters, it is not possible to infer by calculations the maximum, minimum or average amount of NH 3 with high temporal resolution. However, we conducted thermodynamic calculations with the E-AIM (Extended Aerosol Inorganics Model) model [56] , [57] to provide an estimate of the order of magnitude of NH 3 mixing ratios present near Alert during July and August ( Supplementary Fig. 4 ). In July–August at Alert, measurements indicate that average daily temperatures are typically 0–10 °C, and relative humidity is typically between 74 and 82%. We use these ranges of temperature and relative humidity as inputs to the E-AIM model. Meng and Seinfeld [58] indicate that the timescale for equilibration depends strongly on the particle diameter, and the uptake coefficient for the gas-phase substance. Recent summertime ground, aircraft and ship-based measurements in the Canadian Arctic Archipelago indicate that the particles are predominantly smaller than 100 nm in diameter (favouring fast equilibration), but also significantly neutralized (slowing equilibration timescales by decreasing the uptake coefficient). Recent ship-based observations in the Canadian Arctic Archipelago by Wentworth et al . [14] , found significantly more ammonia in the gas phase than the particle phase over most of the region. Bird colonies represent concentrated sources of NH 3 to the model atmosphere, which likely equilibrates the particles with this new burden of ammonia quickly in the downwind direction. In our simulations, this may lead to slight underestimates of the true mixing ratios of gas-phase ammonia, and slight overestimates of particle-phase ammonium within the first few hours of transport from the source. Even though more neutralized particles take longer to equilibrate, a large increase in gas-phase ammonia will only have a moderate impact on their chemical composition (since they are nearly neutralized), so model predictions assuming equilibrium will not result in large errors. Given that any biases related to assumptions of equilibrium partitioning would cause a low bias in gas-phase ammonia throughout the region, this suggests that our model estimate provides a lower bound on the potential impact of seabird colonies on particle formation. Seabird ammonia emissions Seabirds have a nitrogen-rich diet consisting primarily of marine biota. A significant portion of this nitrogen is excreted in the form of uric acid (C 5 H 4 O 3 N 4 ), which undergoes bacterial degradation in the presence of water (H 2 O) and oxygen (O 2 ) to release carbon dioxide (CO 2 ) and NH 3 , according to the reaction shown in equation 1 (ref. 20 ). The emission inventory for seabird-derived NH 3 used in this work was adapted from a global inventory that Riddick et al . [18] , [19] developed of NH 3 emissions from decomposing seabird guano for over 30,000 different seabird colonies. The foundation of the inventory is a bioenergetics model developed by Wilson et al . [59] , [60] that calculates species-dependent NH 3 emissions per bird. Riddick et al . [18] , [19] used seabird-colony population data from a wide variety of sources to scale up NH 3 emissions to the colony level with a global resolution of 0.1° × 0.1°. The inventory is publically available for download [19] . The original inventory provided three different scenarios each containing a different temperature-dependency for NH 3 volatilization from seabird guano. Here we adopt scenario 3 (moderate dependency), which was identified as being the most accurate by Riddick et al . [18] Riddick et al . [18] discuss the large uncertainties and lack of standard reporting methods for seabird-colony populations. Population uncertainties are magnified for remote regions (that is, the Arctic) where data on seabird populations are sparse. Hence, the Circumpolar Seabird Data Portal (CSDP) [30] was used to check for any substantial seabird colonies in the region north of 50° N that were not included in the Riddick et al . inventory [18] , [19] . The CSDP [30] is an interactive map that displays total seabird population by species in hexagonal cells (roughly 100 km across). The total population in each cell was recorded and transformed into an NH 3 emission estimate using the bioenergetics model [59] , [60] . The emission estimates for each cell in the CSDP were cross-referenced against the Riddick et al . [18] , [19] inventory with the same methodology as used by Wentworth et al . [14] . For colonies in the region north of 50° N that were present in both inventories, the NH 3 emission estimates typically agreed within a factor of 2 (data not shown). Using this methodology, we identified 42 colonies in the region north of 50° N either absent or with significantly lower estimates in Riddick et al . [18] , [19] . The locations and magnitude of annual NH 3 emissions of these extra colonies are listed in the Supplementary Tables 3–5 . These additional colonies contributed about 7.6 Gg NH 3 to the total annual emissions of about 35.6 Gg NH 3 in the region north of 50° N. Although the CSDP is a ‘work in progress’ and may contain errors, it is currently the best available resource for examining Arctic seabird-colony population at the regional scale. Future studies should focus on constraining the uncertainties in Arctic seabird distribution. GEOS-Chem-TOMAS model description The GEOS-Chem-TOMAS chemical-transport model [7] , [28] , [29] ( www.geos-chem.org ) includes a detailed oxidant–aerosol tropospheric chemistry mechanism and is used in the interpretation of the atmospheric measurements. Here we describe the model and additional details are in Supplementary Methods . We use GEOS-Chem version 9-02 at 2° × 2.5° resolution globally, and with 47 vertical layers between the surface and 0.01 hPa. The assimilated meteorology is taken from the NASA Global Modelling and Assimilation Office Goddard Earth Observing System (GEOS-5). Our simulations use 2011 meteorology and allow a 2-month spin-up. In this study, we implemented into GEOS-Chem-TOMAS a total of 35.6 Gg per year of seabird-colony NH 3 emissions, all in the region north of 50° N (28 Gg per year following the Riddick et al . inventory [18] , [19] combined with additional seabird-colony emissions of 7.6 Gg per year derived using seabird population estimates from the Circumpolar Seabird Data Portal [30] and the bioenergetics model of Wilson et al . [59] ). The total seabird-colony NH 3 emissions for the region north of 50° N (35.6 Gg year) used in our simulations are within the range of the emissions scenarios for this region (18 to 37 Gg per year) that was identified by Riddick et al . [18] , [19] . To reflect the migratory pattern of circumpolar seabirds, we distributed the annually averaged emissions evenly between 15 May and 15 September [61] , [62] , [63] . The peaks in NH 3 emissions from seabird colonies may follow episodes of rain [20] , but we have insufficient information to parameterize that process at this time. Implementation of this updated seabird-colony emissions inventory into GEOS-Chem in two previous studies found greater model-measurement consistency for 2014 surface-layer NH 3 (ref. 14 ) and reasonable agreement with summertime-mean aerosol size distributions at Alert, Nunavut, Canada [7] . In addition to the seabird-colony emissions, our simulations include other natural and anthropogenic NH 3 emissions [64] . Paulot et al . [22] , [65] recently evaluated the GEOS-Chem reduced nitrogen simulation and found that the GEOS-Chem model is more likely to overestimate than underestimate the traditional reduced nitrogen sources from the central United States and the Arctic Ocean. Biomass-burning emissions are from the Global Fire Emissions Database v3 (ref. 66 ). The model also includes natural and anthropogenic sources of sulfur dioxide [27] and oceanic DMS concentrations from Lana et al . [67] . Oxidation of SO 2 occurs in clouds by reaction with H 2 O 2 and O 3 and in the gas phase with OH. DMS oxidation occurs by reaction with OH and NO 3 . The TOMAS microphysics scheme is coupled to the GEOS-Chem model and tracks the number and mass of particles within each of 15 dry-size sections [29] . The first 13 size sections are logarithmically spaced, and include aerosol dry diameters from approximately 3 nm to 1 μm, and two additional size sections represent aerosol dry diameters from 1 to 10 μm. Growth and loss of particles with diameters smaller than 3 nm are approximated in the model. The model includes particle growth by condensation of sulfuric acid, organic vapours and MSA. Our simulations include a biogenic secondary organic aerosol source ( ∼ 19 Tg per year) and also enhanced secondary organic aerosol (100 Tg per year), spatially correlated with anthropogenic CO emissions that is considered non-volatile following D’Andrea et al . [68] D’Andrea et al . [68] also explored uncertainties related to the Kelvin effect on retardation of early growth of the particles and found a minor impact on CCN globally. Simulated size-resolved aerosol constituents are sulfate-nitrate-ammonium, sea-spray, hydrophilic organics, hydrophobic organics, internally mixed black carbon, externally mixed black carbon, dust and water. The sulfate–nitrate–ammonium chemistry uses the ISORROPIA II thermodynamic model [69] . Aerosol hygroscopic growth is a function of grid box mean relative humidity capped at 99%. The model includes removal of gases and aerosols from the atmosphere by precipitation, both in and below clouds [70] , as well as by dry deposition using a resistance in-series approach [71] . Wet deposition is an important sink process for aerosols larger than about 50–100 nm in diameter. The model implements wet removal updates developed by Wang et al . [72] to account for wet removal in mixed-phase and ice clouds. In addition, we use the updated aerosol wet removal scheme developed by Croft et al . [7] that includes revisions to the wet removal efficiency and precipitation fraction parameterizations to better represent the efficiency of aerosol scavenging, particularly in the low-clouds of the Arctic. The aerosol in-cloud wet removal in GEOS-Chem-TOMAS is specific to the aerosol size range that is assumed activated into cloud hydrometeors, and includes release of particles back to the atmosphere by evaporation of hydrometeors. Atmospheric Cluster Dynamics Code description The Atmospheric Cluster Dynamics Code (ACDC) [35] , [36] was implemented in the GEOS-Chem-TOMAS (GCT) model for this study. ACDC is a state-of-the-science ternary H 2 SO 4 –NH 3 –H 2 O particle formation scheme [35] , [36] . ACDC is briefly described here and further details are in the Supplementary Methods . The formation rate of particles at circa 1.2 nm in mass diameter is determined from a full kinetics simulation by ACDC model using particle evaporation rates based on quantum chemistry. The approach is driven entirely by these physicochemical interactions, and its behaviour is not fit to ambient or laboratory observations. The formation rate results of hundreds of ACDC runs, varying sulfuric acid concentrations (10 4 –10 9 cm −3 ), ammonia vapour concentrations (10 6 –10 11 cm −3 ), relative humidity (0–100%), temperature (180–320 K) and condensation (scavenging) sink on existing aerosol surface area (10 −5 –10 −1 s −1 ), were systematically recorded in a comprehensive lookup table for use in the GCT model. With this method, we achieve predictions of ternary formation rates more in line with the original ACDC theoretical model, with only a minor additional computational cost. The newly formed particles added to the GCT model have a diameter of 1.2 nm, corresponding to the size for which the ACDC formation rates were calculated. The model has been compared with laboratory observations obtained in the CLOUD (Cosmics Leaving OUtdoor Droplets) chamber [9] . It successfully reproduced, with unparalleled quantitative performance, the H 2 SO 4 –NH 3 formation rates across a broad range of ammonia and sulfuric acid gas-phase concentrations. The capability of ACDC to reproduce the observed formation rates is particularly impressive considering that it was not trained to any of the observation data; the model is entirely governed by the aforementioned collision, evaporation and scavenging rate calculations. Recently, the ACDC-based lookup table has also been used in a regional-scale chemical transport model simulation over Europe and evaluated against both ground site and aircraft measurements from the surface up to 10 km (ref. 36 ). The predicted number concentrations agree reasonably well with the measurements resulting in only a slight over-prediction of particles larger than 4 nm. However, it should be noted that in a transport model set-up, the particle formation scheme is only one factor among many (including, for example, condensation, coagulation, wet and dry deposition schemes) affecting the particle size distribution evolution, and the agreement between predicted and observed particle numbers is expected to improve as further improvements to the description of the aerosol microphysics are implemented [36] . Calculation of cloud-condensation nuclei concentrations As an additional evaluation of our Arctic simulations, we calculated the cloud-condensation nuclei at 0.2% super saturation (CCN0.2) based on the simulated aerosol number and mass distributions and compared with summertime measurements from the inner Arctic, north of 80° N [3] . We calculated the effective hygroscopicity parameter (κ) using the composition of each model size bin and then determined the total number of aerosols that could activate at 0.2% supersaturation based on κ-Kohler theory [73] . We chose this supersaturation to match available measurements. However, supersaturations in the pristine Arctic environment could easily reach 0.6% or larger and thus CCN0.2 should not be considered as an exact proxy for cloud-droplet number. Calculation of Arctic EL-VOC-based particle formation rates We also conducted calculations to evaluate the possibility of EL-VOCs to contribute to particle formation rates in the Arctic. We use recently presented measurement data for the Arctic Ocean, which indicates an air–sea flux of 0.27–0.78 μg m −2 d −1 for monoterpenes [74] . Using the maximum air–sea flux and assuming a yield of 0.03 for EL-VOCs, we find the EL-VOC rate in units of g m −2 s −1 : We also assume a boundary layer height of 100 m and a condensation sink of 3.43 × 10 −4 s −1 and calculate EL-VOC concentration: We then apply the equation (2) of Riccobono et al . [75] to parameterize the particle formation rate as a function of sulfuric acid and ELVOC: We use a typical H 2 SO 4 concentration from our summertime simulations at Alert of 5 × 10 6 cm −3 and calculate J =0.03 s −1 . Such a low particle formation rate suggests that typical EL-VOC levels near Alert are likely not sufficient to yield appreciable particle formation, although we cannot rule out their additional contributions. Certainly low-volatility marine organics are expected to play an important role in particle growth and their size-resolved sources in the Arctic are associated with a high degree of uncertainty [74] . Although our simulations are generally consistent with the current state of knowledge, organic emissions are highly uncertain and not well size resolved for the Arctic [76] . Missing low-volatility organics could suppress particle growth in our simulations, yielding an underestimate of the growth to sizes that act as the seeds for cloud-droplet formation. Alternatively missing primary organic aerosol emissions could suppress particle growth through acting as a greater condensation sink. The role of organics in particle formation and growth in the Arctic is an important subject for future research. Calculation of CDNC We make an offline calculation of the CDNC using monthly averaged aerosol number and mass concentrations from our GEOS-Chem-TOMAS simulations. We use the activation parameterization of Abdul-Razzak and Ghan [77] . We assume aerosol constituents are mixed internally within each size bin, and calculate the hygroscopicity parameter, κ, as a volume weighted average of the individual aerosol constituents [73] . We assume a constant updraft velocity of 0.5 m s −1 for the results presented in Fig. 5a . We examined the maximum supersaturation achieved with an updraft velocity of both 0.1 and 0.5 m s −1 at the model level corresponding to approximately 915 hPa ( Supplementary Fig. 8 ). Assuming an updraft velocity of 0.1 m s −1 results in a maximum supersaturation in the Arctic region of 0.15–0.25%, while increasing this updraft to 0.5 m s −1 results in a noticeably higher supersaturation (in the range of 0.3–0.5%), both within a reasonable range for the summertime Arctic. We also examined the corresponding minimum critical diameters for activation at each updraft velocity ( Supplementary Fig. 9 ). To do this, we used a constant κ of 0.4 as a simplifying assumption, to yield about the minimum aerosol size that could activate to form a cloud droplet based on our simulations. However, our full method used to produce the CDNC values presented in Fig. 5a calculates κ for each size bin in each model grid box based on the aerosol composition. These minimum critical diameters range from 80 to 110 nm for the 0.1 m s −1 updraft and 40 to 80 nm for the 0.5 m s −1 updraft. Calculation of aerosol-induced cloud-albedo radiative effect To estimate the aerosol-induced cloud-albedo radiative effect (also termed the aerosol indirect effect or AIE), we calculate the change in top-of-the-atmosphere radiation using an offline version of the Rapid Radiative Transfer Model for GCMs [78] , [79] . Monthly averaged cloud fraction, temperature, pressure and cloud liquid-water content are from NASA GEOS5 meteorology fields. We first assume a control cloud drop radius of 10 microns and then perturb this value by taking the ratio of the simulated number of activated particles with and without NH 3 emissions from seabird guano, to the one-third power [48] , [49] . We assume constant cloud liquid-water content for the control and perturbed simulations, such that changes in cloud-droplet number are associated with changes in cloud-droplet radius, and thus changes in cloud optical depth. The above methodology is used to calculate the aerosol indirect (cloud-albedo) effect presented in Fig. 5b . Methodology for exploring uncertainties in AIE We conducted sensitivity studies to examine the potential impact of uncertainties related to ammonia emissions, MSA, primary organic aerosols and assumptions about cloud updraft velocity on the cloud-albedo radiative effects attributed to seabird-colony ammonia emissions. We examined the effects of both doubling and halving all seabird-colony ammonia emissions (simulations 2xNH3 and 0.5xNH3, respectively). In another sensitivity study, we assumed that MSA behaved the same as sulfate and acted along with sulfate in particle formation (simMSA). In addition, we conducted a sensitivity study assuming a constant flux of primary organic aerosol from the ocean of 2.84 μg m −2 per day following Browse et al . [80] (simPOA). Finally, we conducted two sensitivity studies with updraft velocities of 0.1 and 1.0 m s −1 (simvel0.1 and simvel1.0, respectively). Some of these uncertainties can strengthen (2xNH3, simMSA, simvel1.0), whereas others can weaken (0.5xNH3, simPOA, simvel0.1) the indirect effect relative to our standard simulation. Supplementary Table 2 shows that these factors could yield uncertainty of about a factor of two in our calculated pan-Arctic mean aerosol indirect effect. Future work is needed to improve knowledge related to these uncertainties so that better model parameterizations can be developed. Code availability The GEOS-Chem-TOMAS model used in this study is freely available for download from www.geos-chem.org . To derive the results presented in this study, additional code modifications to the wet scavenging and particle formation parameterizations are necessary. Additional off-line post-processing scripts are required as well to calculate the changes in cloud properties and radiative effects. This additional code is available from corresponding authors upon request. The E-AIM Model II is accessible online at ( http://www.aim.env.uea.ac.uk/aim/model2/model2a.php ). The seabird-colony ammonia emissions data that were implemented in the GEOS-Chem-TOMAS model are freely available in the NERC Environmental Information Data Centre with the identifier doi:10.5285/c9e802b3-43c8-4b36-a3a3-8861d9da8ea9 . Additional seabird-colony ammonia emissions data are available from the Circumpolar Seabird Data Portal at http://axiom.seabirds.net/maps/js/seabirds.php . Data availability The findings in this study are based on model output from the GEOS-Chem-TOMAS model and measurement data. Requests for the model output can be sent to B.C. (betty.croft@dal.ca), and requests for measurement data can be sent to G.R.W. (greg.wentworth@gov.ab.ca) and W.R.L. (richard.leaitch@canada.ca). How to cite this article: Croft, B. et al . Contribution of Arctic seabird-colony ammonia to atmospheric particles and cloud-albedo radiative effect. Nat. Commun. 7, 13444 doi: 10.1038/ncomms13444 (2016). Publisher's note: Springer Nature remains neutral with regard to jurisdictional claims in published maps and institutional affiliations.